Local BMP receptor activation at adherens junctions in theDrosophilagermline stem cell niche According to the stem cell niche synapse hypothesis postulated for the mammalian haematopoietic system, spatial specificity of niche signals is maximized by subcellularly restricting signalling to cadherin-based adherens junctions between individual niche and stem cells. However, such a synapse has never been observed directly, in part, because tools to detect active growth factor receptors with subcellular resolution were not available. Here we describe a novel fluorescence-based reporter that directly visualizes bone morphogenetic protein (BMP) receptor activation and show that in the Drosophila testis a BMP niche signal is transmitted preferentially at adherens junctions between hub and germline stem cells, resembling the proposed synapse organization. Ligand secretion involves the exocyst complex and the Rap activator Gef26, both of which are also required for Cadherin trafficking towards adherens junctions. We, therefore, propose that local generation of the BMP signal is achieved through shared use of the Cadherin transport machinery. We study stem cell niche interactions in the Drosophila testis, where the hub, a group of somatic niche stromal cells, is surrounded both by germline stem cell (GSCs) and somatic stem cells called cyst stem cells (CySCs). Two key niche signals contribute to the maintenance of GSC fate. First, hub cells secrete the cytokine-like growth factor Upd that activates the Jak/Stat signalling cascade through its receptor Dome [1] , [2] . As loss of Upd signalling leads to GSC loss by premature differentiation, it was initally thought that this pathway directly controls GSC stemness [3] . However, recent observations suggest that the effect of Upd on GSC fate is at least in part mediated indirectly through Jak/Stat activation in the somatic CySCs. Indeed, GSC maintenance is sensitive to depletion of the Stat92E transcription factor or its targets chinmo or Zfh-1 in somatic cells of the testis [4] , [5] , [6] , whereas loss of Jak/Stat activity in GSCs primarily affects adhesion to the hub [6] . The second GSC niche signal is mediated by the bone morphogenetic protein (BMP) ligands Dpp and Gbb [7] , [8] . As in the ovary [9] , activation of the BMP pathway in the male germline directly represses transcription of the differentiation factor bam in GSCs and their immediate progeny, the gonialblasts [7] , [10] . This is the key determinant for the maintenance of GSC stemness, because ectopic Bam expression in GSCs is sufficient to induce stem cell loss [8] , [11] through premature differentiation [12] . BMP growth factors are expressed by both the hub and other somatic cells including the CySCs [7] . It is therefore important to address the relative contributions of either source to the BMP niche signal. In the absence of artificial somatic Jak/Stat pathway overactivation [4] , [5] that secondarily induces increased BMP signalling in the germline [6] , only GSCs in direct contact with the hub cells maintain stem cell fate. Consequently, GSCs begin to express Bam and lose stem cell fate when they are displaced from the hub following a loss of Cadherin-mediated adhesion [13] , [14] or are outcompeted by CySCs with increased adhesiveness [15] . Thus, a direct BMP signal from the hub cells is likely to be required for GSC maintenance. Because Dpp expression levels are increased in hub cells in comparison with other somatic cells [7] , this signal is presumably mediated by Dpp or Dpp/Gbb heterodimers [7] , [16] . Consistently, the niche signal strictly requires the Dpp-specific type I BMP receptor Tkv, and ectopic overexpression of Dpp but not Gbb is able to cause full repression of bam transcription [7] . The contact dependence of the niche signals is surprising, given that BMP growth factors are normally acting over much larger distances. However, according to the stem cell niche synapse hypothesis [17] , [18] , communication within the mammalian bone marrow haematopoietic niche is restricted to individual stem and stromal cells by organizing niche signalling around N-cadherin based junctions. Correspondingly, we hypothesized that a similar cadherin-based synapse between individual hub cells and GSCs might direct transmission of the BMP niche signals to specific germline cells, thus restricting signal range. However, this could not be adressed using existing assays for BMP pathway activation, for example, phospho-SMAD immunostaining [19] , that impart no subcellular spatial information about where on the plasma membrane signals are received. We, therefore, developed a fluorescence-based reporter capable of detecting activated BMP receptors with subcellular resolution, and confirmed that BMP niche signals from the hub are received at discrete sites on the GSC surface associated with adherens junctions. A fluorescence based reporter for BMP receptor activation The inhibitor protein FKBP12 specifically binds to the unphosphorylated GS (glycine-serine rich) domain of inactive type I BMP receptors, blocking the kinase domain [20] . GS domain phosphorylation by the type II receptor following ligand binding displaces FKBP12 and generates a binding site for the R-Smad transcription factor. This inhibitor to substrate binding switch defines the activated state of the receptor [21] . We attached a genetically encoded reporter cassette consisting of the conformation sensitive circularly permutated yellow fluorescent protein (cpYFP) core of the InversePericam Ca 2+ sensor [22] and FKBP12 (the reporter is hence abbreviated as TIPF for Tkv-InversePericam-FKBP12) to the Drosophila type I BMP receptor Tkv. Analogous to the Ca 2+ -mediated interaction of the InversePericam amino- and carboxy-terminal domains, FKBP12 binding to inactive Tkv should suppress cpYFP fluorescence, whereas its displacement following phosphorylation should allow the cpYFP core to adopt a fluorescent conformation ( Fig. 1a ) while making the phosphorylated GS domain available for signalling. We confirmed that the reporter retains receptor function by rescuing the lethality of amorphic tkv alleles in transgenic flies ubiquitously expressing TIPF ( Supplementary Table S1 ). 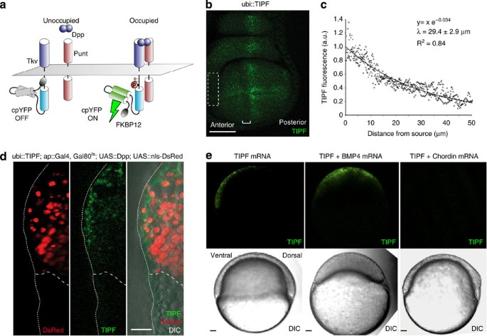Figure 1: TIPF is a fluorescent reporter for BMP receptor activation. (a), Intramolecular interaction between FKBP12 (black) and the unphosphorylated GS domain of the inactive type I BMP receptor Tkv (blue) forces the InversePericam cpYFP core into a nonfluorescent conformation (grey). On receptor activation GS domain phosphorylation (red) displaces FKBP12 and allows the cpYFP to adopt a fluorescent state. (b), In live ubi∷TIPF wing discs, reporter fluorescence (green) forms a gradient in both anterior and posterior compartments, dipping along the compartment boundary. This pattern accurately presages Mad phosphorylation. Image Z projection of the most apical 5 μm. (c), Normalized TIPF fluorescence plotted against distance from the compartment boundary (a.u., arbitrary units). Different symbols denote individual discs, black curve exponential fit to average of all discs. Fluorescence decays exponentially with a decay length (29.4±2.9 μm) comparable with GFP–Dpp and pMad gradients. (d), TIPF fluorescence in ubi∷TIPF; ap∷Gal4 tub∷Gal80ts; UAS∷Dpp/UAS∷nls-DsRed discs. Dpp overexpression following a 4 h heat shock at 30 °C leads to an increase in TIPF fluorescence (green) in the dorsal compartment (border outline by dashed lines) where ap∷Gal4 is active as shown by nuclear DsRed fluorescence (red). Imaged area approximately corresponding to area of low endogenous signalling marked by dashed box in (b,e), Zebrafish embryos injected withDrosophilaTIPF mRNA. Reporter fluorescence (green) is present on the presumptive ventral side where endogenous BMP signalling is active. Shield formation (arrowhead) demarcates the dorsal side. Coinjection of BMP4 mRNA expands the domain of TIPF fluorescence and ventralizes the embryo. Chordin overexpression dorsalizes the embryo and abolishes TIPF fluorescence. Scale bars 50 μm except (d), 10 μm. Figure 1: TIPF is a fluorescent reporter for BMP receptor activation. ( a ), Intramolecular interaction between FKBP12 (black) and the unphosphorylated GS domain of the inactive type I BMP receptor Tkv (blue) forces the InversePericam cpYFP core into a nonfluorescent conformation (grey). On receptor activation GS domain phosphorylation (red) displaces FKBP12 and allows the cpYFP to adopt a fluorescent state. ( b ), In live ubi ∷ TIPF wing discs, reporter fluorescence (green) forms a gradient in both anterior and posterior compartments, dipping along the compartment boundary. This pattern accurately presages Mad phosphorylation. Image Z projection of the most apical 5 μm. ( c ), Normalized TIPF fluorescence plotted against distance from the compartment boundary (a.u., arbitrary units). Different symbols denote individual discs, black curve exponential fit to average of all discs. Fluorescence decays exponentially with a decay length (29.4±2.9 μm) comparable with GFP–Dpp and pMad gradients. ( d ), TIPF fluorescence in ubi ∷ TIPF; ap ∷ Gal4 tub ∷ Gal80 ts ; UAS ∷ Dpp/UAS ∷ nls-DsRed discs. Dpp overexpression following a 4 h heat shock at 30 °C leads to an increase in TIPF fluorescence (green) in the dorsal compartment (border outline by dashed lines) where ap ∷ Gal4 is active as shown by nuclear DsRed fluorescence (red). Imaged area approximately corresponding to area of low endogenous signalling marked by dashed box in ( b , e ), Zebrafish embryos injected with Drosophila TIPF mRNA. Reporter fluorescence (green) is present on the presumptive ventral side where endogenous BMP signalling is active. Shield formation (arrowhead) demarcates the dorsal side. Coinjection of BMP4 mRNA expands the domain of TIPF fluorescence and ventralizes the embryo. Chordin overexpression dorsalizes the embryo and abolishes TIPF fluorescence. Scale bars 50 μm except ( d ), 10 μm. Full size image To validate our reporter, we turned to the larval wing disc, where BMP pathway activity is quantitatively well understood [23] . TGF-β signalling responds largely linearly to ligand concentration [24] , TIPF should be activated in a graded manner in the wing disc, reflecting the Dpp morphogen gradient and presaging the phospho-SMAD pattern. Consistently, in live L3 discs TIPF fluorescence ( Fig. 1b ) decreased exponentially with increasing distance from the Dpp producing domain. The decay length of this gradient (29.4±2.9 μm, Fig. 1c ) was roughly comparable with published values for the ligand (17.0±6.5 μm or 22.5±6.5 μm) [25] , [26] and downstream phospho-SMAD gradients (25.2±4.5 μm) [26] , [27] . Reporter fluorescence was increased in domains ectopically overexpressing Dpp and adjacent receiving cells ( Fig. 1d ) and abolished by RNAi-mediated knockdown [28] of the type II receptor Punt that drives Tkv phosphorylation ( Supplementary Fig. S1a–c ). BMP receptors function as oligomeric complexes containing multiple type I subunits even before ligand exposure [29] . Thus, TIPF fluorescence exhibited a local minimum along the compartment boundary ( Fig. 1b ) reflecting the local drop in BMP pathway activation caused by Hh dependent repression of endogenous tkv [19] , although ubi ∷ TIPF expression itself is uniform ( Supplementary Fig. S1d ). As vertebrate and fly BMP pathway components are at least partially compatible [30] , we also tested the TIPF reporter in developing zebrafish embryos to further validate the detection principle. In gastrulating vertebrate embryos BMP pathway activation defines the ventral side [31] . Consistently, when synthetic messenger RNA, encoding the TIPF reporter, was injected at the single-cell stage, reporter fluorescence was in the majority of embryos (65.2%, n =46, Supplementary Table S2 ) confined to the ventral body half around shield stage, when dorsoventral assymmetry can first be detected morphologically. This region of reporter activation was expanded when BMP4 mRNA was coinjected, and reduced or abolished by overexpression of the BMP inhibitor Chordin ( Fig. 1e ). Junction-associated BMP receptor activation in the GSC niche We next expressed our reporter in the fly germline under control of the nos ∷ Gal4VP16 driver. Fluorescence could be detected in conspicuous punctate regions of high signal intensity at the interface between GSCs and hub cells indicating strong local receptor activation ( Fig. 2a ; Supplementary Fig. S2 for schematic description of image planes). However, BMP receptor overexpression is known to cause ligand independent pathway activation [32] . Thus, in testis expressing the TIPF reporter under nos ∷ Gal4VP16 control, we observe background pathway activation around all germ cells ( Fig. 2a ), and equivalent overexpression of a Tkv–Cherry fusion protein causes tumour-like accumulations of immature germ cells ( Supplementary Fig. S3a ). To ascertain that the punctate signals at the GSC/hub interface correspond to BMP ligands locally released by the hub cells, we therefore expressed the TIPF reporter directly from a weaker, germline-specific promotor, avoiding the amplification step inherent to the Gal4 system. We chose a truncated version of the Bam promotor from which the sequences responsible for BMP-dependent repression in the GSCs were deleted and which had previously been shown to drive GFP expression in all early germ cells in the ovary [9] . This construct (BamΔ27 ∷ TIPF) drives moderate reporter expression in the germ cells of the testis tip including the GSCs ( Fig. 2b,c ). Since TIPF fluorescence does not withstand the permeabilization required for GFP antibody staining, we combined detection of the receptor signal with anti-Tkv immunostaining against the extracellular portion of both TIPF and endogenous Tkv. Reporter fluorescence and hence Tkv activation in BamΔ27 ∷ TIPF testes was limited to small, subcellular foci at the interface between hub cells and GSCs and, therefore, associated with only a subset of the total receptor pool. Extra, presumably inactive receptors were detected elsewhere on the GSC cortex, within the hub, and in differentiating germ cells ( Fig. 2d ), resembling the overall distribution of endogenous Tkv ( Supplementary Fig. S3b ). Reception of the BMP niche signal is thus limited to subcellular foci on the GSC surface facing the hub, although receptors are in principle more widely available. 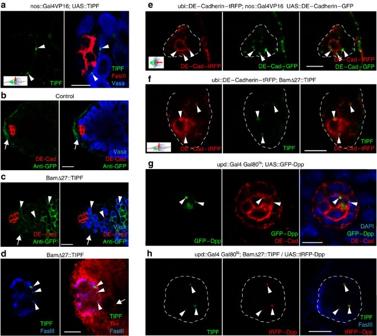Figure 2: BMP signalling in the testis GSC niche. (a), TIPF expression in the germline under nos∷Gal4-VP16 control. Strong reporter fluorescence (green) is detected in small foci on the hub cell / GSC interface (arrrowheads). Germline cells labelled by Vasa (blue), hub cells with FasIII (red). (b,c) The BamΔ27 promoter fragment drives TIPF in the germline. (b), In control testes GFP antibody staining (green) produces background in the somatic muscle sheath (arrow). (c), In BamΔ27∷TIPF testes, reporter expression can be detected in germ cells from GSCs to cyst stages with increasing intensity (arrowheads, hub marked by DE–Cadherin in red). (d), BMP signalling is spatially restricted. In a central section through a BamΔ27∷TIPF testis tip reporter fluorescence (green, arrowheads) is limited to subcellular foci on the interface between GSCs and hub cells marked by FasIII (blue). The total Tkv pool is detected by immunostaining (red) elsewhere on the GSCs (arrow) and throughout the gonad. (e), Distinct junctions connect hub cells and GSCs. In optical sections through the hub/GSC interface, DE–Cadherin–GFP (green) expressed in the germline under nos∷Gal4VP16 control co-localizes (arrowheads) with punctate concentrations of DE–Cadherin–RFP expressed in somatic cells from the ubi promoter, but not with the apical junctional belt connecting adjacent hub cells. (f), Receptor activation coincides with hub/GSC junctions. In live BamΔ27∷TIPF; ubi∷DE–Cadherin–RFP testes, TIPF fluorescence (green, arrowheads) coincides with the punctate adherens junctions between hub and GSCs marked by DE–Cadherin–RFP (red). (g), GFP–Dpp (green, arrowheads) expressed in the hub co-localizes with adherens junctions marked by DE–Cadherin immunostaining (red). Apical transverse section, DNA (DAPI) in blue. (h), Receptor activation reflects local ligand accumulation. In upd∷Gal4, tub∷Gal80ts; UAS∷tagRFP–Dpp / BamΔ27∷TIPF flies, reporter fluorescence in the germline (green) coincides with local concentrations of tagRFP–Dpp (red, arrowheads) in underlying hub cells (marked by FasIII, blue, central section). Orientation of image planes in (a–d) and (e–h) indicated by small insets, see also suppl.Fig. 2a. Scale bars 5 μm except (b,c) 10 μm. Figure 2: BMP signalling in the testis GSC niche. ( a ), TIPF expression in the germline under nos ∷ Gal4-VP16 control. Strong reporter fluorescence (green) is detected in small foci on the hub cell / GSC interface (arrrowheads). Germline cells labelled by Vasa (blue), hub cells with FasIII (red). ( b , c ) The BamΔ27 promoter fragment drives TIPF in the germline. ( b ), In control testes GFP antibody staining (green) produces background in the somatic muscle sheath (arrow). ( c ), In BamΔ27 ∷ TIPF testes, reporter expression can be detected in germ cells from GSCs to cyst stages with increasing intensity (arrowheads, hub marked by DE–Cadherin in red). ( d ), BMP signalling is spatially restricted. In a central section through a BamΔ27 ∷ TIPF testis tip reporter fluorescence (green, arrowheads) is limited to subcellular foci on the interface between GSCs and hub cells marked by FasIII (blue). The total Tkv pool is detected by immunostaining (red) elsewhere on the GSCs (arrow) and throughout the gonad. ( e ), Distinct junctions connect hub cells and GSCs. In optical sections through the hub/GSC interface, DE–Cadherin–GFP (green) expressed in the germline under nos ∷ Gal4VP16 control co-localizes (arrowheads) with punctate concentrations of DE–Cadherin–RFP expressed in somatic cells from the ubi promoter, but not with the apical junctional belt connecting adjacent hub cells. ( f ), Receptor activation coincides with hub/GSC junctions. In live BamΔ27 ∷ TIPF; ubi ∷ DE–Cadherin–RFP testes, TIPF fluorescence (green, arrowheads) coincides with the punctate adherens junctions between hub and GSCs marked by DE–Cadherin–RFP (red). ( g ), GFP–Dpp (green, arrowheads) expressed in the hub co-localizes with adherens junctions marked by DE–Cadherin immunostaining (red). Apical transverse section, DNA (DAPI) in blue. ( h ), Receptor activation reflects local ligand accumulation. In upd ∷ Gal4, tub ∷ Gal80 ts ; UAS ∷ tagRFP–Dpp / BamΔ27 ∷ TIPF flies, reporter fluorescence in the germline (green) coincides with local concentrations of tagRFP–Dpp (red, arrowheads) in underlying hub cells (marked by FasIII, blue, central section). Orientation of image planes in ( a – d ) and ( e – h ) indicated by small insets, see also suppl. Fig. 2a . Scale bars 5 μm except ( b , c ) 10 μm. Full size image Do these sites of signal transduction correspond to adherens junctions, as postulated by the stem cell niche synapse hypothesis? We generated a ubi ∷ DE–Cadherin–RFP transgene that in control epithelia faithfully labels adherens junctions ( Supplementary Fig. S4a ). Because the ubiquitin promotor has low germline activity ( Supplementary Fig. S4b ) in the testis, this construct most strongly marks the apical belts of adherens junctions connecting neighbouring somatic hub cells ( Fig. 2e,f ). In addition, punctate concentrations of cadherins become apparent in apical transverse sections across the top of the hub cells, overlapping with or just adjacent to this apical belt ( Fig. 2e–g ). We could not distinguish the two junction populations based on differences in their complement of intracellular junction components ( Supplementary Fig. S5a ), although a similar discontinuous distribution had been reported for GFP-tagged Par-3 (ref. 6 ). Instead, we juxtaposed the somatic DE–Cadherin–RFP with DE–Cadherin–GFP expressed in germline. Whereas the belt of adherens junctions between hub cells was marked by RFP alone, the punctate junctions were labelled by both GFP and RFP and thus correspond to adherens junctions connecting GSCs and hub cells ( Fig. 2e ; Supplementary Fig. S5b,c ). In testes carrying both the BamΔ27 ∷ TIPF and ubi ∷ DE–Cadherin–RFP constructs, receptor activation in the GSCs coincided with the punctate adherens junctions between hub and GSCs ( Fig. 2f ). At the same time, GFP–Dpp expressed in the hub was localized apically, at or just below the junctional level, again largely co-localizing with the punctate adherens junctions facing the GSCs ( Fig. 2g ). Correspondingly, in testes expressing the TIPF reporter in the germline and a functional tagRFP–Dpp fusion protein ( Supplementary Fig. S6 ) in the hub, BMP receptor activation in the GSCs coincided with the local concentrations of ligand in the underlying hub cells ( Fig. 2h ). Thus, in keeping with the stem cell niche synapse hypothesis, the BMP niche signal is transduced locally at the junctions between stem and niche cells. Generation of the local BMP niche signal Transmission of ovary or testis niche signals is affected when DE–Cadherin in GSCs is mutated [33] , downregulated [6] , or its trafficking impaired [13] . RNAi mediated knockdown under upd ∷ Gal4 Gal80 ts control removed DE–Cadherin from the hub ( Fig. 3a,b ). However, germ cells abutting the hub maintained stem-cell state as shown by bam repression ( Fig. 3a,b ) and the presence of punctate spectrosomes ( Fig. 3c,d ). In addition, armadillo was still recruited to the junctions in the absence of DE–Cadherin ( Fig. 3b ), presumably due to the continued presence of DN-Cadherin ( Fig. 3c,d ). Because reduction of Cadherin on the hub side equally affects adhesion to all GSCs and CySCs, no single population gained a competitive advantage allowing it to displace its neighbours [15] . DE–Cadherin protein as such is therefore not essential for correct niche signalling. 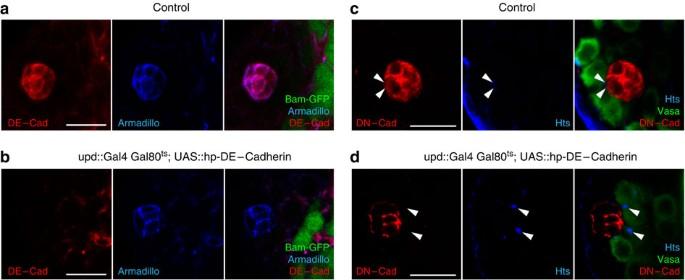Figure 3: RNAi mediated knockdown of DE–Cadherin in the hub. (a), In controls lacking the DE–Cadherin RNAi hairpin transgene, the hub is marked by DE–Cadherin (red) and armadillo (blue). Bam∷GFP (green) is excluded from germline cells contacting the hub. (b), Knockdown of DE–Cadherin under upd∷Gal4, Gal80tscontrol (5 days induction at 30 °C) abolishes DE–Cadherin in the hub. Armadillo recruitment andBamrepression are not affected. (c), In control flies, DN-Cadherin marks adherens junctions in the hub (red). Germ cells (marked by Vasa, green) contacting the hub are GSCs and posses punctate spectrosomes stained by 1B1/anti-Hts (red). (d), Following DE–Cadherin knockdown in the hub, DN-Cadherin remains at the junctions, and the germ cells contacting the hub retain stem cell fate. Scale bars=10 μm. Figure 3: RNAi mediated knockdown of DE–Cadherin in the hub. ( a ), In controls lacking the DE–Cadherin RNAi hairpin transgene, the hub is marked by DE–Cadherin (red) and armadillo (blue). Bam ∷ GFP (green) is excluded from germline cells contacting the hub. ( b ), Knockdown of DE–Cadherin under upd ∷ Gal4, Gal80 ts control (5 days induction at 30 °C) abolishes DE–Cadherin in the hub. Armadillo recruitment and Bam repression are not affected. ( c ), In control flies, DN-Cadherin marks adherens junctions in the hub (red). Germ cells (marked by Vasa, green) contacting the hub are GSCs and posses punctate spectrosomes stained by 1B1/anti-Hts (red). ( d ), Following DE–Cadherin knockdown in the hub, DN-Cadherin remains at the junctions, and the germ cells contacting the hub retain stem cell fate. Scale bars=10 μm. Full size image In Drosophila pupal [34] and embryonic epithelia [35] , cadherins are transported to the adherens junctions through the recycling endosome (RE) and exocyst-dependent secretory/recycling vesicles. Loss of exocyst function traps cadherins in enlarged Rab11-positive REs. Because exocyst-tagged vesicles are themselves recruited to adherens junctions by β-catenin [34] , a positive feedback loop polarizes DE–Cadherin membrane transport towards existing adherens junctions. Similar mechanisms also operate in mammalian cells [36] , [37] . To verify that this trafficking machinery is also involved in junction formation and maintenance in the hub, we expressed transgenic RNAi constructs [28] against several exocyst complex members (Sec5, Sec6, Sec8, Sec10, Sec15, Exo70) using a upd ∷ Gal4 tub ∷ Gal80 ts driver. Of these, only constructs directed against the core exocyst components Sec6 and Sec8 caused detectable, consistent phenotypes. We therefore limited further analysis to these two complex members. Following exocyst knockdown, transmembrane adhesion molecules like DE–Cadherin ( Fig. 4a,b ) or Fasciclin III ( Supplementary Fig. S7a ) accumulated within the hub cells. As expected [34] , [35] , internalized DE–Cadherin co-localized with a massively enlarged Rab11-positive recycling compartment ( Fig. 4c,d ; Supplementary Fig. S7b ). In consequence, with increasing duration of exocyst knockdown, the hub progressively lost its compact tissue organization ( Fig. 4a,d ), ultimately disintegrating into isolated cells ( Fig. 4b , Supplementary Fig. S7a ). This hub disintegration was not associated with increased apoptosis of hub cells ( Supplementary Fig. S7c ). 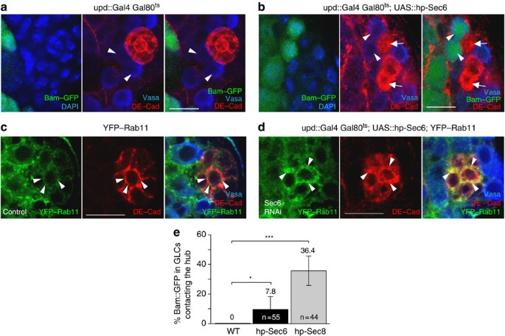Figure 4: Exocyst complex involvement in cadherin trafficking in the hub. (a,b), Exocyst function is required for hub integrity. (a), Control testes have compact hubs marked by DE–Cadherin (red). Bam∷GFP fluorescence (green) is absent from GSCs (arrowheads, germline marked by Vasa, blue). (b), Transgenic Sec6 RNAi driven by upd∷Gal4 Gal80ts. DE–Cadherin accumulates within detaching hub cells (arrows), while GSCs begin to express Bam∷GFP. (c,d), Sec6 knockdown traps DE–Cadherin in the recycling compartment. (c), In control testes, DE–Cadherin is concentrated at junctions (red, arrowheads), overlapping only weakly with REs marked by YFP–Rab11 (green). Germ cells marked with Vasa (blue). (d), Following Sec6 knockdown, hub cells show increased YFP–Rab11 fluorescence and DE–Cadherin relocates from junctions to enlarged Rab11-positive endosomes (arrowheads). (e) Germline cells begin expressing Bam while still contacting hub cells (Sec6: 7.8%,P=0.0229,n=55; Sec8: 21.5%,P=0.00041,n=44, Fisher's exact test). Images central sections, scale bars 10 μm, error bars denote s.d. Controls subjected to induction regimes of respective experiments. Figure 4: Exocyst complex involvement in cadherin trafficking in the hub. ( a , b ), Exocyst function is required for hub integrity. ( a ), Control testes have compact hubs marked by DE–Cadherin (red). Bam ∷ GFP fluorescence (green) is absent from GSCs (arrowheads, germline marked by Vasa, blue). ( b ), Transgenic Sec6 RNAi driven by upd ∷ Gal4 Gal80 ts . DE–Cadherin accumulates within detaching hub cells (arrows), while GSCs begin to express Bam ∷ GFP. ( c , d ), Sec6 knockdown traps DE–Cadherin in the recycling compartment. ( c ), In control testes, DE–Cadherin is concentrated at junctions (red, arrowheads), overlapping only weakly with REs marked by YFP–Rab11 (green). Germ cells marked with Vasa (blue). ( d ), Following Sec6 knockdown, hub cells show increased YFP–Rab11 fluorescence and DE–Cadherin relocates from junctions to enlarged Rab11-positive endosomes (arrowheads). ( e ) Germline cells begin expressing Bam while still contacting hub cells (Sec6: 7.8%, P =0.0229, n =55; Sec8: 21.5%, P =0.00041, n =44, Fisher's exact test). Images central sections, scale bars 10 μm, error bars denote s.d. Controls subjected to induction regimes of respective experiments. Full size image However, maintenance of GSC stemness was strongly affected in the exocyst knockdown testes. We observed bam derepression indicating a loss of BMP niche signalling not only in isolated germ cells, but also in germline cells still attached to hub cells losing Sec6 (7.3%, n =55 cells, Fig. 4b,e ) or Sec8 function (36.4%, n =44 cells, Fig. 4e; Supplementary Fig. S7a ), suggesting that BMP pathway activity in GSCs was lost before detachment from the hub. Interfering with the cadherin-trafficking machinery in ligand-producing cells therefore affects niche function before the receiving cells drift out of signal range [13] , [14] , [33] . Strikingly, mutations in Gef26 / dizzy , an activator of the small GTPase Rap1 that is involved in junction maintenance [38] , also affect both cadherin localization in the hub and niche signalling [14] . We, therefore, wondered whether Dpp might share the trafficking machinery used by DE–Cadherin for targeted delivery to the plasma membrane, as this would intrinsically entail local ligand secretion at the junctions. Consistent with an involvement of the exocyst complex in Dpp secretion, GFP–Dpp [39] in hub cells co-localized strongly with vesicles marked by either Sec15 immunostaining ( Fig. 5a) or a functional Sec15–Cherry fusion protein (74.4±26.0% of GFP–Dpp punctae, n =102, Supplementary Fig. S8a ; Supplementary Table S3 ). Association with Sec5 carrying vesicles was less pronounced ( Supplementary Fig. S8b,c ). 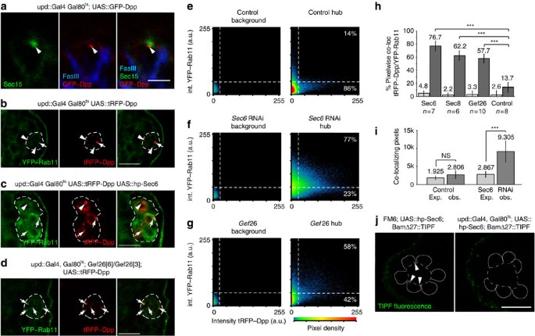Figure 5: Exocyst complex involvement in Dpp signalling in the hub. (a), GFP–Dpp (green) expressed under upd∷Gal4, tub∷Gal80tscontrol co-localizes with local, apical concentrations of the exocyst component Sec15 (red). Hub cells (marked with FasIII, blue). (b–d), Co-localization of tagRFP–Dpp expressed in the hub by upd∷Gal4, tub∷Gal80tswith YFP–Rab11.b, In control testes, few tRFP-Dpp (red) punctae coincide (arrow) with Rab11 endosomes (green), while most do not (arrowheads). In Sec6 RNAi (c) andGef263/ Gef266mutant (d) testes, co-localization becomes more common. (e–g), Pixelwise quantification of Dpp / Rab11 co-localization. Intensity in the green (YFP–Rab11) channel is plotted against tRFP-Dpp fluorescence, heat map indicates pixel density. (e), In control testes 86% of tRFP-Dpp positive pixels are below background for YFP–Rab11 (bottom right quadrant). In Sec6 RNAi testes (f) 77% and inGef26mutant testes (g) 58% of tRFP-Dpp pixels are double positive (upper right quadrant). (h,i), Quantification of RNAi effects. (h), Exocyst knockdown orGef26 mutation significantly increases pixelwise co-localization of tagRFP–Dpp with YFP–Rab11 in hub cells (dark grey bars, light grey bars indicate background, 6–10 replicates/class, ANOVA followed by Tukey's HSD,P<0.0001) (i), The observed co-localization (obs.) between tRFP-Dpp and YFP–Rab11 is significantly increased relative to the value expected for random distribution of positive pixels (exp.) following Sec6 RNAi (Student'st-test,t=3.75,P=0.0006,n=6) but not in control testes (t=1.65,P=1.376,n=6). (j), Exocyst RNAi suppresses BMP signalling. TIPF fluorescence (green) at the GSC-hub interface of control flies (arrowheads) is abolished by Sec6 knockdown. Scale bars 10 μm except (a), 2 μm. Images central sections, dashed outlines mark hub, solid outlines GSC boundaries, error bars denote s.d. Controls subjected to induction regimes of respective experiments. Figure 5: Exocyst complex involvement in Dpp signalling in the hub. ( a ), GFP–Dpp (green) expressed under upd ∷ Gal4, tub ∷ Gal80 ts control co-localizes with local, apical concentrations of the exocyst component Sec15 (red). Hub cells (marked with FasIII, blue). ( b – d ), Co-localization of tagRFP–Dpp expressed in the hub by upd ∷ Gal4, tub ∷ Gal80 ts with YFP–Rab11. b , In control testes, few tRFP-Dpp (red) punctae coincide (arrow) with Rab11 endosomes (green), while most do not (arrowheads). In Sec6 RNAi ( c ) and Gef26 3 / Gef26 6 mutant ( d ) testes, co-localization becomes more common. ( e – g ), Pixelwise quantification of Dpp / Rab11 co-localization. Intensity in the green (YFP–Rab11) channel is plotted against tRFP-Dpp fluorescence, heat map indicates pixel density. ( e ), In control testes 86% of tRFP-Dpp positive pixels are below background for YFP–Rab11 (bottom right quadrant). In Sec6 RNAi testes ( f ) 77% and in Gef26 mutant testes ( g ) 58% of tRFP-Dpp pixels are double positive (upper right quadrant). ( h , i ), Quantification of RNAi effects. ( h ), Exocyst knockdown or Gef 26 mutation significantly increases pixelwise co-localization of tagRFP–Dpp with YFP–Rab11 in hub cells (dark grey bars, light grey bars indicate background, 6–10 replicates/class, ANOVA followed by Tukey's HSD, P <0.0001) ( i ), The observed co-localization (obs.) between tRFP-Dpp and YFP–Rab11 is significantly increased relative to the value expected for random distribution of positive pixels (exp.) following Sec6 RNAi (Student's t -test, t =3.75, P =0.0006, n =6) but not in control testes ( t =1.65, P =1.376, n =6). ( j ), Exocyst RNAi suppresses BMP signalling. TIPF fluorescence (green) at the GSC-hub interface of control flies (arrowheads) is abolished by Sec6 knockdown. Scale bars 10 μm except ( a ), 2 μm. Images central sections, dashed outlines mark hub, solid outlines GSC boundaries, error bars denote s.d. Controls subjected to induction regimes of respective experiments. Full size image Although the exact molecular role of Gef26 function in DE–Cadherin secretion is unclear, we also tested whether exocyst RNAi or Gef26 / dizzy mutations could trap Dpp in Rab11-positive REs. In contrast to the striking expansion of the YFP–Rab11Rab11-positive recycling compartment caused by knockdown of either Sec6 ( Fig. 5b,c ) or Sec8 ( Supplementary Fig. S9a ) in the hub, reduction of Gef26 levels using two different mutant allele combinations caused moderately increased YFP–Rab11 fluorescence in all cells of the testis ( Fig. 5d ; Supplementary Fig. S9b ). We quantified co-localization of Dpp and Rab11 in the hub as the fraction of tagRFP–Dpp positive pixels that were in single confocal slices also positive for YFP–Rab11 ( Fig. 5e–g ; Supplementary Fig. S9c,d ). The average pixelwise co-localizations in exocyst knockdown and Gef26 mutant testes were significantly increased in comparison with sibling controls ( Fig. 5h ; controls 13.7±2.6%, n =8; Sec6 RNAi 76.7±7.4%, n =7; Sec8 RNAi 62.2±7.2%, n =6; Gef26 3 /Gef26 6 57.7±6.6%, n =10, P <0.0001, one way analysis of variance (ANOVA) with Tukey's HSD). To exclude that this increased overlap was a false positive effect caused by the diffuse expansion of YFP–Rab11, we verified that the observed increase in pixelwise co-localization following Sec6 RNAi was significantly larger than expected for random co-localization ( Fig. 5i ). For the same reason, we sampled co-localization in all genetic backgrounds exclusively at local maxima of the tagRFP–Dpp and YFP–Rab11 distributions, obtaining similarly increased co-localization fractions ( Supplementary Fig. S10 ; see Methods for details). The altered intercellular Dpp distribution was associated with the loss of the BMP niche signal, as TIPF fluorescence was lost from GSCs abutting the hub ( Fig. 5j ) even after short periods of exocyst knockdown (24 h) that did not yet visibly affect tissue integrity. We therefore conclude that exocyst function is required for generation of the Dpp signal in the hub, and that Dpp secretion involves trafficking through the recycling compartment, either directly or via a reinternalization step. In the fly wing disc [23] or the early vertebrate embryo [31] , BMPs spread across dozens of cell diameters forming long-range morphogen gradients. In contrast, in the testis BMP pathway activity, as measured by bam repression, is limited to GSCs, gonialblasts, and two cell cysts, that is, a range of two-to-three cell diameters from the hub. Because Gbb-mediated signalling from somatic cyst progenitor and cyst cells is at least partly responsible for bam repression in the early differentiating germ cells [7] , it is unclear whether the Dpp signal from the hub even reaches that far. We, therefore, wondered whether Dpp secreted from the hub formed a steep gradient dropping below the threshold for bam repression within these two or three cell diameters, or whether alternatively the junction-associated signal transduction implied contact dependent signalling restricted to neighbouring cells. As BMP-signalling range is highly sensitive to changes in ligand production when growth factors can freely move through the tissue [23] , and germ cells distant from the hub can respond to ectopic Dpp [7] , [8] , increased ligand production in the hub should in the first case be able to extend the range of bam repression. We overexpressed Dpp in the hub under control of the upd ∷ Gal4 Gal80 ts driver, using a lacZ reporter for the positively regulated BMP target gene dad as a readout for pathway activation. In control flies, β-Gal protein was present in GSCs and early differentiating germ cells (gonialblasts and early cysts) at roughly equal levels ( Fig. 6a ), presumably due to both Gbb signalling and β-Gal protein perdurance [7] . Following a 4 h pulse of Dpp overexpression in the hub, GCS exhibited elevated β-Gal levels in comparison with gonialblasts and early cysts, indicating that Dpp signalling as such was increased ( Fig. 6b ). However, even continuing Dpp overexpression for up to five days did not increase the range of bam repression ( Fig. 6c,d ). Thus, Dpp produced in the hub locally signals to the adjacent GSCs, but seems to be unable to spread throughout the testis tip ( Fig. 6e ). 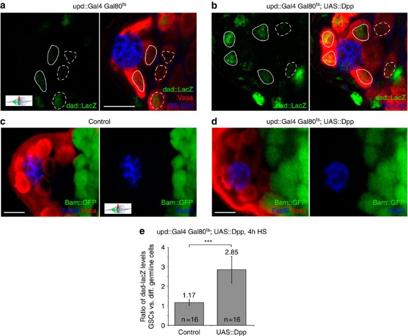Figure 6: The testis niche BMP signal is range restricted. (a,b), BMP pathway activation by GFP–Dpp overexpression in the hub. (a), In control flies, endogenous Dpp signalling is reflected by a transcriptional reporter for the Dpp target genedad(dad∷lacZ, green). Levels in GSCs (solid outlines) and differentiating germ cells (dashed) are comparable (hub marked by DE–Cadherin, red, germ cells by Vasa, blue). (b), Following a 4 h heat shock, dad∷lacZ levels are increased in GSCs of upd∷Gal4, tub∷Gal80ts; UAS∷Dpp / dad∷lacZ flies relative to germ cells further from the hub. (c), In wild-type testes Bam∷GFP reporter transcription (green) in germ cells (Vasa, red) starts roughly two cells from the hub (FasIII, blue). (d), Dpp overexpression in the hub under upd∷Gal4, tub∷Gal80tscontrol for 5 days has no effect on the range ofBamrepression. (e), Quantification of Dpp overexpression effects in dad∷lacZ levels. In control flies (no UAS∷Dpp), average dad∷lacZ levels in GSCs and early differentiating germ cells from the same fly are comparable. Dpp overexpression in the hub increases pathway activity in GSCs relative to differentiating germ cells (n=16 samples/class,t=4.85,P<0.0001, Student'st-test). Scale bars 5 μm, all images single central sections, error bars denote s.d. Figure 6: The testis niche BMP signal is range restricted. ( a , b ), BMP pathway activation by GFP–Dpp overexpression in the hub. ( a ), In control flies, endogenous Dpp signalling is reflected by a transcriptional reporter for the Dpp target gene dad (dad ∷ lacZ, green). Levels in GSCs (solid outlines) and differentiating germ cells (dashed) are comparable (hub marked by DE–Cadherin, red, germ cells by Vasa, blue). ( b ), Following a 4 h heat shock, dad ∷ lacZ levels are increased in GSCs of upd ∷ Gal4, tub ∷ Gal80 ts ; UAS ∷ Dpp / dad ∷ lacZ flies relative to germ cells further from the hub. ( c ), In wild-type testes Bam ∷ GFP reporter transcription (green) in germ cells (Vasa, red) starts roughly two cells from the hub (FasIII, blue). ( d ), Dpp overexpression in the hub under upd ∷ Gal4, tub ∷ Gal80 ts control for 5 days has no effect on the range of Bam repression. ( e ), Quantification of Dpp overexpression effects in dad ∷ lacZ levels. In control flies (no UAS ∷ Dpp), average dad ∷ lacZ levels in GSCs and early differentiating germ cells from the same fly are comparable. Dpp overexpression in the hub increases pathway activity in GSCs relative to differentiating germ cells ( n =16 samples/class, t =4.85, P <0.0001, Student's t -test). Scale bars 5 μm, all images single central sections, error bars denote s.d. Full size image Exocyst involvement in long-range BMP signalling To test whether exocyst-dependent secretion is unique for the short-range Dpp signal in the hub, we looked at the fly wing disc. In. contrast to the hub, GFP–Dpp in wing disc epithelial cells coincided only weakly with Sec15–Cherry (2.3±0.3%, n =284, Fig. 7a ), indicating differences in the dynamics of intracellular trafficking between these tissues ( Supplementary Fig. S11a,b ). Nevertheless, GFP–Dpp accumulated within expanded Rab11-positive REs in clones of Dpp-producing cells lacking the core exocyst subunit Sec5 (37.7±9.2% of GFP–Dpp punctae, n =169) relative to heterozygous sibling (14.2±5.9%, n =305) or wild-type cells (12.8±5.1%, n =586, Fig. 7b,c ; Supplementary Fig. S12 ). As expected [34] , [35] , the enlarged REs in Sec5 clones also accumulated DE–Cadherin (56.1±13.0%, n =450) in comparison with those in heterozygous control tissue (20.2±3.6%, n =582, Fig. 7c,d ; Supplementary Fig. S13 ). As in the hub, Dpp in the wing disc therefore requires exocyst function for export from the recycling compartment. Consistently, the exocyst complex and the Dpp pathway interact genetically: Reducing Sec15 copy number partially rescued the pupal lethality caused by Gal4-mediated overexpression of GFP–Dpp in its endogenous domain in the wing disc ( Fig. 8a ; Supplementary Table S4 ). RNAi-mediated reduction of the core exocyst component Sec6 in all Dpp producing cells lead to growth retardation of the disc (diameter 200.2±19.0 μm versus 230.4±20.8 μm in controls, Student's t -test P <0.0001) and a narrowing of the expression domain of the high-level target gene Sal (width 52.8±8.8 μm versus 69.5±6.5 μm in controls, Student's t -test P =0.00042), indicating reduced Dpp activity ( Fig. 8b,c ). 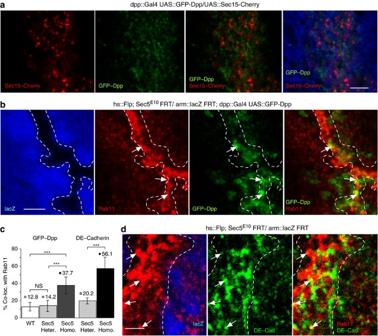Figure 7: The exocyst complex is involved in cadherin and Dpp trafficking in the wing disc. (a), GFP–Dpp (green) and Sec15–Cherry (red) show low levels of co-localization in wing disc epithelial cells outlined with FasIII (blue). (b), GFP–Dpp mislocalization to REs in Sec5 clones. In larval wing discs, GFP–Dpp expressed under dpp∷Gal4 control (green, (b), apical section) accumulates in enlarged REs marked by Rab11 immunostaining (red, arrows) within Sec5 mutant clones also lacking β-Gal immunostaining (blue), but not in heterozygous tissue within the same disc (arrowheads). (c), Quantification of cargo mislocalization. In Sec5 clones, the fraction of GFP–Dpp found in the Rab11 compartment (dark grey,n=169) is increased relative to wild-type (white,n=586,t=7.8,P<0.0001) or heterozygous sibling cells (light grey,n=305,t=6.55,P<0.0001, Student'st-test). The fraction of DE–Cadherin co-localizing with Rab11 (black,n=450) in Sec5 clones is similarly increased in comparison to control sibling cells (grey,n= 582,t=5.97,P=0.00028, Student'st-test). (d), DE–Cadherin (green, optical section below junctional level) accumulates in Rab11 positve REs in Sec5 mutant clones marked by the absence of β-Gal immunostaining (blue) relative to adjacent heterozygous cells. Scale bars (a), 25 μm, (b,c), 5 μm, error bars denote s.d. Figure 7: The exocyst complex is involved in cadherin and Dpp trafficking in the wing disc. ( a ), GFP–Dpp (green) and Sec15–Cherry (red) show low levels of co-localization in wing disc epithelial cells outlined with FasIII (blue). ( b ), GFP–Dpp mislocalization to REs in Sec5 clones. In larval wing discs, GFP–Dpp expressed under dpp ∷ Gal4 control (green, ( b ), apical section) accumulates in enlarged REs marked by Rab11 immunostaining (red, arrows) within Sec5 mutant clones also lacking β-Gal immunostaining (blue), but not in heterozygous tissue within the same disc (arrowheads). ( c ), Quantification of cargo mislocalization. In Sec5 clones, the fraction of GFP–Dpp found in the Rab11 compartment (dark grey, n =169) is increased relative to wild-type (white, n =586, t =7.8, P <0.0001) or heterozygous sibling cells (light grey, n =305, t =6.55, P <0.0001, Student's t -test). The fraction of DE–Cadherin co-localizing with Rab11 (black, n =450) in Sec5 clones is similarly increased in comparison to control sibling cells (grey, n = 582, t =5.97, P =0.00028, Student's t -test). ( d ), DE–Cadherin (green, optical section below junctional level) accumulates in Rab11 positve REs in Sec5 mutant clones marked by the absence of β-Gal immunostaining (blue) relative to adjacent heterozygous cells. Scale bars ( a ), 25 μm, ( b , c ), 5 μm, error bars denote s.d. 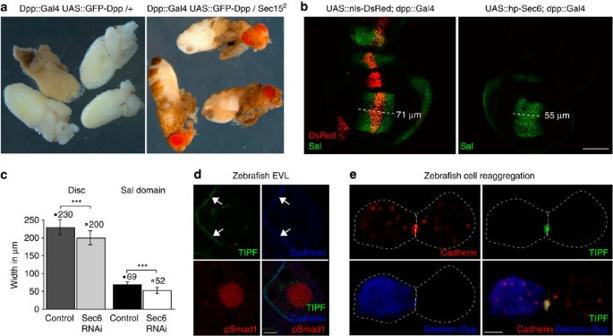Figure 8: BMP signalling in the wing disc and the zebrafish embryo. (a), Sec15 genetically interacts with the Dpp pathway. At 25 °C, Dpp∷Gal4 UAS∷GFP–Dpp larvae overexpressing GFP–Dpp in the endogenous domains of the imaginal discs manage to pupariate but arrest shortly after disc eversion. Removal of one functional copy of Sec15 allows development to proceed to pharate adult stage with rare hatching escapers. (b), Exocyst RNAi knockdown suppresses Dpp morphogen signalling. Following a 48 h heat shock at 29 °C, UAS∷hpSec6/+; dpp∷Gal4 Gal80ts/+ L3 wing discs are smaller and have a narrower expression domain of the high level Dpp target gene Sal (green) when compared with age-matched UAS∷nls-DsRed/+; dpp∷Gal4 Gal80ts/+ controls. (c), Quantification of the Sec6 RNAi effect. Wing disc diameter (light grey,n=13 discs) and Sal domain width (white,n=8) are reduced following Sec6 RNAi in Dpp producing cells (controls dark grey,n=19 and black,n=8, Student'st-testt=4.97,P<0.0001 andt=3.51,P=0.00042, respectively). (d), In Zebrafish EVL cells with active BMP signalling as shown by pSmad1 immunostaining (red), cortical TIPF fluorescence (green, arrows) is restricted to cell boundaries that also harbour Cadherin (blue). (e), In reaggregating cell pairs from dissociated zebrafish embryos injected either with TIPF or Dpp mRNA (marked by Dextran tracer, blue), TIPF fluorescence (green) co-localizes with the reforming adherens junctions (red). Scale bars (b), 50 μm, (d,e), 5 μm. Error bars denote s.d. Full size image Figure 8: BMP signalling in the wing disc and the zebrafish embryo. ( a ), Sec15 genetically interacts with the Dpp pathway. At 25 °C, Dpp ∷ Gal4 UAS ∷ GFP–Dpp larvae overexpressing GFP–Dpp in the endogenous domains of the imaginal discs manage to pupariate but arrest shortly after disc eversion. Removal of one functional copy of Sec15 allows development to proceed to pharate adult stage with rare hatching escapers. ( b ), Exocyst RNAi knockdown suppresses Dpp morphogen signalling. Following a 48 h heat shock at 29 °C, UAS ∷ hpSec6/+; dpp ∷ Gal4 Gal80 ts /+ L3 wing discs are smaller and have a narrower expression domain of the high level Dpp target gene Sal (green) when compared with age-matched UAS ∷ nls-DsRed/+; dpp ∷ Gal4 Gal80 ts /+ controls. ( c ), Quantification of the Sec6 RNAi effect. Wing disc diameter (light grey, n =13 discs) and Sal domain width (white, n =8) are reduced following Sec6 RNAi in Dpp producing cells (controls dark grey, n =19 and black, n =8, Student's t -test t =4.97, P <0.0001 and t =3.51, P =0.00042, respectively). ( d ), In Zebrafish EVL cells with active BMP signalling as shown by pSmad1 immunostaining (red), cortical TIPF fluorescence (green, arrows) is restricted to cell boundaries that also harbour Cadherin (blue). ( e ), In reaggregating cell pairs from dissociated zebrafish embryos injected either with TIPF or Dpp mRNA (marked by Dextran tracer, blue), TIPF fluorescence (green) co-localizes with the reforming adherens junctions (red). Scale bars ( b ), 50 μm, ( d , e ), 5 μm. Error bars denote s.d. Full size image Finally, we returned to the zebrafish model to test whether BMP signals are generated in a similar manner outside the fly system. In the gastrulating fish embryo the enveloping layer (EVL) is partially epithelial in character, and its leading edge cells form adherens junctions with each other and their more animal neighbours [40] . In embryos overexpressing TIPF, reporter fluorescence and hence BMP receptor activation in EVL cells exposed to endogenous BMP signals coincided with the animal and lateral adherens junctions but was absent from the vegetal cell boundary lacking cadherins ( Fig. 8d ). Consistently, when zebrafish embryos were injected with mRNA encoding TIPF or Dpp, dissociated, and the cells mixed and reaggregated, BMP signalling was limited to re-forming adherens junctions between reporter and ligand-expressing cells ( Fig. 8e ). Although we did not analyse the distribution of the exocyst in these cells, it is worth noting that, in mammalian cell lines, exocyst components are also recruited to adherens junctions and thus similarly localize to the incipient junctions when neighbouring cells establish contact [36] , [37] . In summary, we have shown that in keeping with the stem cell niche synapse hypothesis [17] , [18] , a BMP niche signal in the Drosophila testis is transduced at subcellularly confined sites associated with adherens junctions between hub cells and GSCs. Although BMP ligands are also produced by the somatic CySCs, we did not detect BMP receptor activation at the GSC surfaces facing the CySCs. There are several nonexclusive explanations that may contribute to this observation. Either, niche signalling is indeed dominated by the homodimeric Dpp or heterodimeric Dpp/Gbb ligands that are produced preferentially by the hub cells [7] . In support of this idea, Dpp but not Gbb can fully suppress bam transcription upon ectopic expression [7] , and is, at least in the wing, thought to have higher signalling activity [16] . Alternatively, signalling from the CySCs may occur diffusely over the entire GSC surface and thus become diluted below the detection threshold of our reporter. Finally, based on the expression profile of the BMP ligands [7] signalling from the CySCs is presumably dominated by Gbb and may therefore preferentially act through the alternative type I BMP receptor Saxophone [16] , thus avoiding detection by our Tkv-specific reporter. However, without artificial Jak/Stat pathway over-activation in the somatic cells of the testis, the CySC-derived BMP signal is by itself not sufficient to maintain GSC fate. Consequently, GSC detachment form the hub induces Bam derepression [6] indicating a loss of BMP pathway activation [7] , [10] . The junction-associated BMP signal from the hub to the germline, we have described here, is therefore essential for GSC maintenance. In addition, we have shown that trafficking of both Dpp and DE–Cadherin in the hub cells involves the exocyst complex and the Rab11-positive recycling compartment. We propose that the local release of the junctional BMP signal is achieved through this shared use of intracellular machinery. Admittedly, RNAi-mediated inactivation of the exocyst complex is bound to have pleiotropic effects, and we cannot exclude that the secretion of Upd or other growth factors may not also be affected. Can the observed loss of GSC stemness following exocyst knockdown therefore be directly attributed to a loss of BMP signalling from the hub? We believe that this is the case, because loss of Jak/Stat signalling in the germline would primarily be expected to affect adhesion of the GSCs to the hub [6] . Although this loss of contact secondarily causes Bam derepression, we have observed Bam expression also in GSCs still adhering to the hub. As Bam expression indicates a loss of BMP signalling also in the testis [7] , [8] , [10] , we attribute this directly to the loss of the junction-associated BMP signal that we directly detected using our reporter. Future studies are required to address what directs Dpp secretion within the hub cells towards the adherens junctions with the overlying GSCs rather than towards those facing the adjacent hub cells. In addition, we have begun to investigate how the BMP ligands are confined after secretion to prevent lateral diffusion away from the site of release. It is likely that for the latter proteoglycans has an essential role [41] . Finally, we have shown that the exocyst is also required for generation of the Dpp signal in the wing disc, where it forms a long-range morphogen gradient rather than a contact-dependent niche signal. It will be interesting to test whether this reflects a specific requirement of planar transcytosis [39] , with the junctions forming a two dimensional network of signalling synapses. Alternatively, as suggested by the zebrafish experiments, subcellularly restricted signal transduction at intercellular junctions may be a more general mechanism operating also in systems where BMP ligands spread through extracellular diffusion [42] . Fly stocks The mutant strains tkv 8 , tkv A12 , Sec15 1 , Sec15 2 , Sec5 E10 , Sec5 E13 , Gef26 3 , Gef26 6 , Gef26 dizzy1 , the Gal4-driver lines upd ∷ Gal4, ap ∷ Gal4, nos ∷ Gal4VP16, hh ∷ Gal4, and dpp ∷ Gal4, and the repressor lines tub ∷ Gal80 and tub ∷ Gal80 ts have all been described (see Flybase for references, http://www.flybase.org ). The following VDRC RNAi lines [28] were used: VDRC37279 (UAS ∷ hp-Put), VDRC22079 (UAS ∷ hp-Sec6), and VDRC45032 (UAS ∷ hp-Sec8), VDRC27081 (UAS ∷ hp-DE–Cadherin). Transgene and plasmid constructs The UAS ∷ GFP–Dpp [39] , UAS ∷ Dpp [43] , tub ∷ YFP–Rab11 (ref. 44 ), and Bam ∷ GFP [9] transgenic lines have been described. UAS ∷ tRFP-Dpp flies were made by replacing the GFP fragment from pCaSpeR-UAS ∷ GFP–Dpp [39] with tagRFP (Evrogen, abbreviated throughout as tRFP). For ubiquitous expression of red fluorescent DE–Cadherin, the tRFP ORF was inserted into pUP-DECH-Nc generating pUP-DECH-tRFP, analogous to pUP-DECH-GFP [45] . Promoter and ORF were then transferred into pCaSpeR4 (ref. 46 ) generating pCaSpeR-Ubi ∷ DE–Cadherin-tRFP. To generate UAS ∷ Sec15–Cherry and UAS ∷ Tkv-Cherry flies, the coding sequences of Sec15 (GenBank nucleotide core accession code 24648622) and Tkv (GenBank nucleotide core accession code 28574651) were PCR amplified from an embryonic cDNA library, cloned into pUAST, and the mCherry ORF [47] inserted C-terminally. For ubiquitous, Gal4-independent expression, the UAS cassette was replaced by the ubiquitin promoter from pUP-DECH-tRFP. The TIPF reporter was generated by joining the cpYFP core from Inverse Pericam [22] and Drosophila FKBP12 (GenBank nucleotide core accession code 1209721) via fusion PCR. This reporter cassette was then C-terminally fused to the Tkv isoform D ORF (GenBank nucleotide core accession code 28574651) via a GTG linker. The finished reporter was then inserted into pUAST [48] generating UAS ∷ TIPF. Replacing the UAS cassette with the ubiquitin promoter from pUP-DECH-NcoI yielded pCaSpeR-Ubi ∷ TIPF. To achieve Gal4-independent germline expression, the UAS promoter was replaced by the Bam promoter and 5′-UTR truncated at the EcoRI site at +27 (BamΔ27 ∷ TIPF), which deleted the GSC-specific silencer element [9] . For zebrafish RNA injections, the Dpp and TIPF ORFs were cloned into the pCS2+ expression vector generating pCS2-Dpp and pCS2-TIPF. Plasmid and PCR primer sequences are available from the authors on request. Transgenic flies were either generated by BestGene or in the lab according to standard protocols. Immunocytochemistry and microscopy Immunostainings procedures of imaginal discs [27] were followed also for testes. Larvae or males were dissected in PEM (80 mM PIPES, 5 mM EGTA, 1 mM MgCl 2, pH 7.4) buffer, samples prefixed with 4% PFA in PEM, fixed with 4% PFA in PEM containing detergent (0.1% Tween-20 if maintenance of TIPF fluorescence was required, otherwise 0.2% Triton X-100), quenched with 50 mM NH 4 Cl in PEM, washed, and blocked with 0.5% BSA. Primary antisera were applied o/n at 4 °C at the following dilutions: Mouse anti FasIII 7G10 (ref. 49 ) (obtained via the DSHB, Bloomington) 1:100, rat anti DE–Cadherin DCAD2 (DSHB, [50] ) 1:100, rabbit anti Vasa [51] 1:10,000, rabbit anti Sec5 (ref. 52 ) 1:1000, mouse anti Sec5 22A2 (ref. 53 ) 1:25 to 1:100, guinea pig anti Sec15 (ref. 54 ) 1:2000, rabbit anti Tkv extracellular domain [55] 1:750, rabbit anti Sal [56] 1:1000, rabbit anti Rab11 (ref. 57 ) 1:1000, mouse anti β-Gal (Promega) 1:1000, chicken anti GFP (Abcam) 1:2500, rabbit anti pan-zfCadherin (Sigma) 1:200, Mouse anti pSMAD1 (Cell Signaling) 1:1000. Secondary antisera (Santa Cruz) were used at 1:500 dilution, and DAPI at 1:10,000. Confocal images were collected using Leica SP5/II, SP5 MP, or Zeiss LSM510 or 780 microscopes using DAPI, GFP, tagRFP, mCherry, YFP, Alexa 488, Alexa 568, and Alexa 633 fluorophores. Images were processed with ImageJ/Fiji (Z projections, cropping, scale bars) and final figures assembled using the Adobe CS4 suite. Deconvolution of multiphoton stacks was performed using the Autoquant package (Media Cybernetics). Confocal images are single sections if not explicitly stated otherwise. Imaging and quantification of TIPF reporter fluorescence For the analysis of the TIPF gradient, wing discs were dissected in clone8 medium [58] , mounted peripodial membrane down in MatTek glass bottom tissue culture dishes, covered in clone8 medium, and imaged on an inverse confocal microscope. For quantification, wing pouch regions were isolated in individual image slices and the resulting stacks maximum intensity Z projected. Hh-dependent downregulation of BMP pathway activation in the producing domain [19] of ubi ∷ TIPF 4-1, tkv 8 /CyO discs provided a marker for the anteroposterior compartment boundary. TIPF fluorescence intensity and distance from the compartment boundary were measured using ImageJ/Fiji in two parallel rectangular regions of interest spanning the posterior compartment (one each on the dorsal and ventral sides). Fluorescence intensity was then background corrected, averaged for each disc, fitted to a single exponential function, and normalized to the fluorescence values of this function at x =0. Imaging and quantification of trafficking phenotypes To inactivate exocyst components or DE–Cadherin in the hub, upd ∷ Gal4, tub ∷ Gal80 ts ; tub ∷ YFP–Rab11 or upd ∷ Gal4, tub ∷ Gal80 ts ; bam ∷ GFP virgins were crossed to males from appropriate second chromosome VDRC hairpin RNAi lines. Where required, these males also carried UAS ∷ tagRFP–Dpp/MKRS. Crosses were maintained at 18 °C until hatching to suppress Gal4 activity, and emerging adults transferred to 30 °C for 5 (DE–Cadherin), 7 (Sec6) or 8 days (Sec8) before dissection to induce RNAi. Siblings exposed to the same treatment but lacking the RNAi transgene served as controls. At these induction times, RNAi-induced exocyst depletion phenotypes had become visible, but apoptosis of hub cells as measured by immunostaining against activated Caspase-3 was not yet increased in the disintegrating hubs. Expression of tagRFP–Dpp in upd ∷ Gal4, tub ∷ Gal80 ts ; Gef26 3 / Gef26 6 ; YFP–Rab11, UAS ∷ tRFP-Dpp and upd ∷ Gal4, tub ∷ Gal80 ts ; Gef26 dizzy1 / Gef26 6 ; YFP–Rab11, UAS ∷ tRFP-Dpp males was induced in the same way. For technical reasons, experiments with clones in the wing dics were performed with Sec5 rather than Sec6 , which are both core complex members indispensable for exocyst function [34] , [35] . Homozygous Sec5 clones in the wing disc were generated by heat shocking w hs ∷ FLP; Sec5 E10 FRT40A/ arm ∷ lacZ FRT40A; dpp ∷ Gal4 UAS ∷ GFP–Dpp first instar larvae for 90 min at 37 °C and then raising them at 18 °C to prevent temperature dependent cell loss of the mutant cells [34] . Co-localization between tRFP-Dpp or DE–Cadherin and YFP–Rab11 was first determined pixelwise, plotting fluorescence intensity in the red (Dpp) against the green (Rab11) channel. Average fluorescence levels from germ cell nuclei that should not contain either protein were used to identify background signals. Co-localization was measured as the fraction of above background tRFP-Dpp positive pixels also positive for YFP–Rab11, equivalent to the unweighted co-localization coefficient. Second, to avoid inadvertent false positive co-localization effects caused by diffuse mislocalization of Rab11, especially in the exocyst knockdown conditions, co-localization was sampled only at local maxima of YFP–Rab11 and tRFP-Dpp fluorescence. For this, red and green channels were individually thresholded in Fiji for maximum variance between classes using the algorithm of Otsu [59] , and the resulting binary bitmaps and their overlap quantified using the Fiji particle analysis tool. Co-localization of GFP–Dpp or DE–Cadherin with Rab11 endosomes in the wing disc was analysed accordingly. Finally, we determined the absolute number and area of YFP–Rab11 and tRFP-Dpp positive pixels for control and Sec6 RNAi testes and calculated the co-localization expected for random distribution of these pixels by multiplying the fractions of positive pixels in each channel within the area of interest. These numbers were then compared with the actual levels of co-localization measured within the same samples. To test for effects of exocyst knockdown on Dpp signal generation in the wing disc, we used transgene mediated RNAi to knockdown Sec6 in the entire producing domain. However, expression of the hpSec6 RNAi construct using the dpp ∷ Gal4 driver leads to early larval death before discs can be analysed. To measure the effect of Sec6 knockdown on Dpp signalling in the disc, we, therefore, suppressed expression of the RNAi constructs until L3 discs had formed using tub ∷ Gal80 ts . UAS ∷ hpSec6/UAS ∷ RedStinger males were crossed to dpp ∷ Gal4, tub ∷ Gal80 ts /TM6B, Tb virgins at 18 °C and flipped in 6 h intervals to generate age-matched clutches. This procedure also circumvented the cell lethality caused by exocyst loss at 25 °C (ref. 34 ). Before dissection, larvae were heatshocked at 29 °C for 48 h to induce Sec6 RNAi. UAS ∷ hpSec6/+; dpp ∷ Gal4 Gal80 ts /+ L3 larvae were identified based on their Tb + , DsRed − phenotype, whereas their Tb + , DsRed + UAS ∷ RedStinger/+; dpp ∷ Gal4 Gal80 ts /+ siblings were selected as age and treatment matched controls. After Sal immunostaining discs were imaged using a Leica DMI4000 fluorescence microscope or a Leica SP5 confocal microscope. Disc size and Sal domain width were measured using Fiji. Quantitative differences between experimental and control conditions were tested for significance using Student's t -test, Fisher's exact test, or one way ANOVA followed by Tukey's HSD post hoc test as appropriate for the sample type (frequency or category data, two or more categories, respectively). Zebrafish mRNA injection experiments All zebrafish experiments were carried out according to the relevant university and state animal welfare regulations. Synthetic mRNAs were generated from pCS2-TIPF, pCS2-Dpp, pCS2-Chordin and pCS2-BMP4 (gifts from M. Brand, Dresden) using the MessageMachine SP6 kit (Ambion). 50 pg of TIPF mRNA and 100 pg of BMP4 or Chordin mRNA per embryo were injected into the cytoplasm at the one cell stage. For the detection of reporter fluorescence, individual embryos were mounted in 1% low melt agarose, manually oriented laterally with the shield in the central plane, and imaged in transverse view using a Zeiss LSM510 inverted confocal microscope. For reaggregation experiments, separate batches of embryos were injected with either 50 pg TIPF mRNA or 100 pg Dpp mRNA with 5% rhodamine–dextran (10 kDa) as tracer. Dechorionated embryos were dissociated at dome stage by incubation in DMEM containing 0.5 mg ml −1 trypsin and 0.2 mg ml −1 EDTA for 5 min at 37 °C followed by gentle shaking. How to cite this article: Michel, M. et al . Local BMP receptor activation at adherens junctions in the Drosophila germline stem cell niche. Nat. Commun. 2:415 doi: 10.1038/nocmms1426 (2011).